Enhancing photoelectrochemical water splitting by combining work function tuning and heterojunction engineering We herein demonstrate the unusual effectiveness of two strategies in combination to enhance photoelectrochemical water splitting. First, the work function adjustment via molybdenum (Mo) doping significantly reduces the interfacial energy loss and increases the open-circuit photovoltage of bismuth vanadate (BiVO 4 ) photoelectrochemical cells. Second, the creation and optimization of the heterojunction of boron (B) doping carbon nitride (C 3 N 4 ) and Mo doping BiVO 4 to enforce directional charge transfer, accomplished by work function adjustment via B doping for C 3 N 4 , substantially boost the charge separation of photo-generated electron-hole pairs at the B-C 3 N 4 and Mo-BiVO 4 interface. The synergy between the above efforts have significantly reduced the onset potential, and enhanced charge separation and optical properties of the BiVO 4 -based photoanode, culminating in achieving a record applied bias photon-to-current efficiency of 2.67% at 0.54 V vs. the reversible hydrogen electrode. This work sheds light on designing and fabricating the semiconductor structures for the next-generation photoelectrodes. Photoelectrochemical cell (PEC) for water splitting is a key technology of the future for hydrogen production [1] , [2] , [3] . Despite the widespread attention that has been received, this technology still has many hurdles to overcome and uncharted territories to explore. Ultimately, the photon to hydrogen conversion efficiency has yet to be increased to such a level that commercial applications could become viable [4] . In the PEC water splitting process, photons are first absorbed by the photoelectrode producing electrons and holes, which are then separated and participated in the hydrogen evolution reaction (HER) on cathode and the oxygen evolution reaction (OER) on anode, possibly with the assistance of a bias voltage [1] . Therefore, one way to enhance the PEC efficiency is to increase the quantum efficiency of photons in a PEC system by improving the efficiencies of light harvesting, charge separation and surface charge transfer [3] , [4] , [5] , [6] , [7] , [8] , [9] , [10] . Another strategy to enhance the PEC efficiency is to minimize the overpotential by reducing the voltage loss related to charge recombination, sluggish surface kinetics, etc. BiVO 4 has received great attention in recent years because it is a promising sustainability-inspired photoanode material for PEC with a suitable band gap for visible light absorption [11] and favorable conduction band edge position (0.1–0.2 V vs. NHE) for H 2 evolution [7] . However, the PEC efficiency at low bias voltages of BiVO 4 photoanode still has much room for improvement [11] , [12] , [13] . In particular, due to the presence of numerous trap states and surface defects as well as the associated surface Fermi-level pinning effect, the BiVO 4 films variously prepared so far are still plagued by the quite low open-circuit photo-voltage when used as photoanodes [11] , [14] , [15] . To address this issue, doped photoanodes, such as W-BiVO 4 , Mo-BiVO 4 , have been fabricated aiming to enhance charge transport and to reduce the charge recombination [11] , [12] , [16] , [17] . Meanwhile, W-BiVO 4 /BiVO 4 , Co 2 O 3 /BiVO 4 , and BiOI/BiVO 4 photoanodes have been developed in the form of so-called homojunctions and heterojunctions to enhance the charge separation in PEC systems [6] , [13] , [18] . Other problems of the BiVO 4 -based photoanode include the still low coverage of the solar spectrum which it is able to harvest as well as the low charge separation efficiency. To address these problems, carbon quantum dots/BiVO 4 and nitrogen doped BiVO 4 photoanodes have been reported showing broadened light absorption range, enhanced light harvesting efficiency, and boosted interfacial charge transfer for PEC water splitting [9] , [18] . As for improving the utilization efficiency of surface charge for oxygen evolution, the combined catalyst/photoelectrode systems, such as FeOOH/BiVO 4 , NiFeO x /BiVO 4 , Co-Pi/BiVO 4 , and NiOOH/FeOOH/BiVO 4 , have been commonly used [7] , [19] , [20] , [21] . Recent efforts have improved the photocurrent density of BiVO 4 based photoanodes for water splitting to nearly 90% of its theoretical value at 1.23 V vs. RHE [22] , [23] . However, the photon to hydrogen conversion efficiency is still far from its theoretical value mainly due to the stagnant carrier transport. Especially when a PEC cell works at low bias, the carrier transport is more susceptible to blockage by any potential barriers in the energy landscape along the carrier passage. Specifically, poor performance at low bias of BiVO 4 based photoanodes led to poor applied bias photon-to-current efficiencies (ABPEs) as reported in some PEC water splitting systems, such as Bi-NiFeO x /BiVO 4 (2.25%) [20] , NiOOH/FeOOH/BiVO 4 (1.75%) [7] , NiO/CoO x /BiVO 4 (1.5%) [11] , NiOOH/FeOOH/N-BiVO 4 (2.2%) [9] . Previously, nanostructures and cocatalysts have been used to promote photocurrents and to minimize onset potentials, respectively [7] , [19] , [20] , [21] . Meanwhile, because C 3 N 4 has a favorable conduction band edge position relative to that of BiVO 4 , a heterojunction between the two could increase the charge separation. Prompted by this expectation, the conjugation of C 3 N 4 with BiVO 4 has received great attention in recent years [24] , [25] , [26] , [27] , [28] . However, before the C 3 N 4 /BiVO 4 junction could efficiently drive the PEC water splitting, new strategies must be developed to elaborate the band structure at the junction to optimize charge separation by minimizing interfacial kinetic barriers and energy losses. In this work, we endeavored to explore such ways to further improve the PEC performance of the BiVO 4 photoanode. First, we systematically studied the effect of Mo doping on the electron band structure of BiVO 4 , and discovered that a moderate Mo doping of BiVO 4 , a low end doping regime that has not been explored before, can increase the photo-voltage of BiVO 4 photoanodes from 0.24 V to ~1 V in 10 s irradiation. Second, to further improve the charge separation efficiency at low bias, we elaborated a cliff like junction between B-C 3 N 4 and Mo-BiVO 4 , for which the band structure of C 3 N 4 was judiciously tuned as well by B doping. With such an elaborated junction, interfacial charge transfer was remarkably enhanced. As the main thread running through this work, we make special efforts to advance our ability to modulate the work functions with a view to toning up the NiFeO x /B-C 3 N 4 /Mo-BiVO 4 photoanodes for PEC water splitting. We have significantly increased the light harvesting efficiency (LHE) of the B-C 3 N 4 /Mo-BiVO 4 photoanode, achieving photocurrent densities of 4.7 mA cm −2 at 0.6 V vs. RHE ( Φ Sep = 79%) and 6 mA cm −2 at 1.23 V vs. RHE ( Φ Sep = 98%) in potassium phosphate buffer (PPB) solution with 0.5 M Na 2 SO 3 hole scavenger (pH 7). When the NiFeO x was anchored on the B-C 3 N 4 /Mo-BiVO 4 photoanode as an OER catalyst layer forming the NiFeO x /B-C 3 N 4 /Mo-BiVO 4 photoanode, we obtained photocurrent densities of 3.85 mA cm −2 at 0.54 V vs. RHE (71% IPCE) and 5.93 mA cm −2 at 1.23 V vs. RHE (92% IPCE) in PPB solution without any hole scavengers such as Na 2 SO 3 (pH 7). Significantly, the NiFeO x /B-C 3 N 4 /Mo-BiVO 4 photoanode has achieved an ABPE up to 2.67% at 0.54 V vs. RHE, which is the highest reported to date and yet, with the lowest biased-voltage, for BiVO 4 -based PEC devices. Characterization of the NiFeO x /B-C 3 N 4 /Mo-BiVO 4 photoanode The XRD patterns collected from BiVO 4 , Mo-BiVO 4 , B-C 3 N 4 /Mo-BiVO 4 , NiFeO x /B-C 3 N 4 /Mo-BiVO 4 prepared on the F-doped SnO 2 conducting glass (FTO), C 3 N 4 and B-C 3 N 4 are shown in Supplementary Fig. 1 . All of the diffraction peaks in the XRD patterns obtained can be well indexed to monoclinic BiVO 4 (JCPDS PDF #75–1866), SnO 2 (JCPDS PDF #41–1445) and graphite-C 3 N 4 (JCPDS PDF #50–1250) [18] , [29] , [30] . As shown in Fig. 1a , the champion photoanode consisted of nanoporous B-C 3 N 4 /Mo-BiVO 4 heterojunctions in tandem with a NiFeO x oxygen evolution catalyst (OEC) layer, which were successfully grown on the FTO substrate. (Supplementary Fig. 2 ) As shown in Fig. 1b–g , signals of Bi, C, O, and Fe elements are clearly observed in a row, suggesting that the newly-coated B-C 3 N 4 has covered the nanoporous Mo-BiVO 4 , and NiFeO x layer has covered the B-C 3 N 4 /Mo-BiVO 4 as the OEC. Figures 1h, i is a typical TEM image and a high-resolution TEM (HRTEM) image of the NiFeO x /B-C 3 N 4 /Mo-BiVO 4 sample, respectively, revealing that the B-C 3 N 4 and Mo-BiVO 4 are crystallized (Fig. 1j, k ) while NiFeO x is non-crystallized (Fig. 1l ). The lattice fringes of 0.325 nm and 0.254 nm are ascribed to the (002) plane [31] of C 3 N 4 and the (020) plane [32] of BiVO 4 , respectively. Fig. 1 Electron microscopic characterization of the NiFeO x /B-C 3 N 4 /Mo-BiVO 4 photoanodes. a Top-view (inset is the magnified image) SEM images of the NiFeO x /B-C 3 N 4 /Mo-BiVO 4 photoanode. b HADDF-STEM image of the NiFeO x /B-C 3 N 4 /Mo-BiVO 4 photoanode and c – f the corresponding STEM-EDS elemental mapping images for Bi, C, O, and Fe, respectively. g Overlay of the elemental mapping images of Fe, C, and Bi. 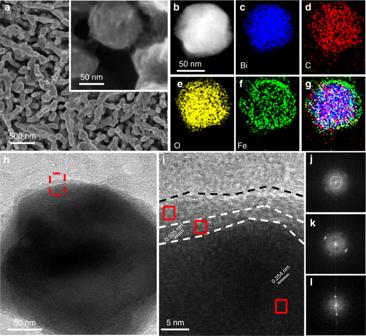Fig. 1 Electron microscopic characterization of the NiFeOx/B-C3N4/Mo-BiVO4photoanodes.aTop-view (inset is the magnified image) SEM images of the NiFeOx/B-C3N4/Mo-BiVO4photoanode.bHADDF-STEM image of the NiFeOx/B-C3N4/Mo-BiVO4photoanode andc–fthe corresponding STEM-EDS elemental mapping images for Bi, C, O, and Fe, respectively.gOverlay of the elemental mapping images of Fe, C, and Bi.hTEM,iHRTEM image of the NiFeOx/B-C3N4/Mo-BiVO4photoanode andj–lcorresponding diffraction patterns via fast Fourier transform of NiFeOx, B-C3N4, and Mo-BiVO4, respectively h TEM, i HRTEM image of the NiFeO x /B-C 3 N 4 /Mo-BiVO 4 photoanode and j – l corresponding diffraction patterns via fast Fourier transform of NiFeO x , B-C 3 N 4 , and Mo-BiVO 4 , respectively Full size image Work function tuning The first strategy we used to optimize the PEC performance of BiVO 4 -based photoanodes, more precisely, to lower the onset potential, was to systematically adjust the work function by Mo doping below 1%, which is a previously uncharted doping regime (the atomic ratio is shown in Supplementary Table 1 ). 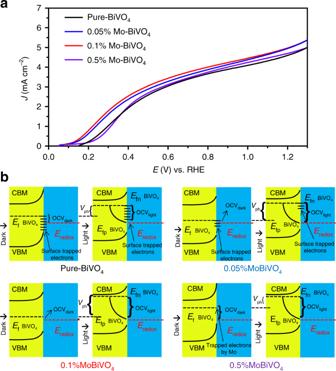Fig. 2 Photoelectrochemical and photo-voltage characterization of the BiVO4-based photoanodes.aLSV curves of pure-BiVO4, 0.05% Mo-BiVO4, 0.1% Mo-BiVO4, and 0.5% Mo-BiVO4recorded at a scan rate of 25 mV s−1under AM 1.5 G one-sun irradiation in PPB solution with 0.5 M Na2SO3as a hole scavenger (pH 7).bBand structures and band bending schematics of pure-BiVO4, 0.05% Mo-BiVO4, 0.1% Mo-BiVO4, and 0.5% Mo-BiVO4, constructed from the XPS, UPS and photoelectrochemical measurement data Figure 2a compares the linear sweep voltammograms (LSV) curves of BiVO 4 (black line), 0.05% Mo doped BiVO 4 (blue line) and 0.1% Mo doped BiVO 4 (red line) 0.5% Mo doped BiVO 4 (purple line) at a scan rate of 25 mV s −1 in 0.5 M Na 2 SO 3 aqueous solution as a hole scavenger with PPB (pH 7) under AM 1.5 G one-sun illumination. The pure BiVO 4 photoanode achieved photocurrent density of 3.2 (±0.3) mA cm −2 at 0.6 V vs. RHE and 4.7 (±0.3) mA cm −2 at 1.23 V vs. RHE, in agreement with the previous report [7] . With a slight doping, the photocurrent density of 0.1% Mo-BiVO 4 increased to 3.4 (±0.2) mA cm −2 at 0.6 V vs. RHE and 4.98 (±0.2) mA cm −2 at 1.23 V vs. RHE. From our extensive measurements, the photocurrent densities assuming 100% absorbed photon-to-current efficiency ( J abs ) of the BiVO 4 -based and the Mo-BiVO 4 -based photoanodes were consistently ~4.7 mA cm −2 and ~5.01 mA cm −2 , respectively (Supplementary Fig. 3 ). The increase in J abs could be ascribed to the enhanced LHE, carrier concentration (Supplementary Fig. 27 ) and mobility (Supplementary Fig. 28 ) resulting from the Mo doping [33] , [34] , [35] , [36] , [37] . More interestingly, the onset potential of Mo doped BiVO 4 (0.05, 0.1, and 0.5%) photoanodes became significantly more negative than that of pure BiVO 4 photoanode, and the rapid photocurrent increase region against bias for the 0.05% and 0.1% Mo doped BiVO 4 is also more negative than that of the BiVO 4 photoanode. However, the rapid photocurrent increase region against bias for the 0.5% Mo doped BiVO 4 is more positive than that of BiVO 4 . This phenomenon is caused by the changed open-circuit photo-voltage (OCP) of BiVO 4 due to the work function adjustment by the Mo doping. Fig. 2 Photoelectrochemical and photo-voltage characterization of the BiVO 4 -based photoanodes. a LSV curves of pure-BiVO 4 , 0.05% Mo-BiVO 4 , 0.1% Mo-BiVO 4 , and 0.5% Mo-BiVO 4 recorded at a scan rate of 25 mV s −1 under AM 1.5 G one-sun irradiation in PPB solution with 0.5 M Na 2 SO 3 as a hole scavenger (pH 7). b Band structures and band bending schematics of pure-BiVO 4 , 0.05% Mo-BiVO 4 , 0.1% Mo-BiVO 4 , and 0.5% Mo-BiVO 4 , constructed from the XPS, UPS and photoelectrochemical measurement data Full size image Supplementary Fig. 5 shows OCP changes of the Mo doped BiVO 4 (0.05, 0.1, and 0.5%) relative to the pure BiVO 4 photoanode due to the truncation of Fermi-level pinning and surface trap states of BiVO 4 . OCP is essentially the difference between open-circuit voltage in dark (OCV dark ) and light (OCV light ). The work function is tuned in such a way that the Fermi level (E f ) is far from CBM when light is off resulting in a small OCV dark , but when light is on (AM 1.5 G), the quasi-Fermi-level (E fn ) becomes as close as possible to CBM giving rise to a large OCV light . Consequently, a large OCP (V ph ) can be obtained. Shown in Supplementary Fig. 5 are the OCP timing profiles of the Mo doped BiVO 4 (0.05, 0.1, and 0.5%) and the pure BiVO 4 photoanodes in PPB solution with the Na 2 SO 3 hole scavenger (pH 7) over a testing interval of 30 s (Supplementary Fig. 5a ) and 2000 s (Supplementary Fig. 5b ). The most important observation is that the 0.1% Mo-BiVO 4 photoanode achieved the highest OCP (~1 V in the first irradiation on/off cycle, and ~0.55 V in the cycles after testing for 1600 s). These OCP values are much higher than those of pure-BiVO 4 (~0.35 V and ~0.15 V), 0.05% Mo-BiVO 4 (~0.8 V and ~0.4 V), and 0.5% Mo-BiVO 4 photoanode (~0.23 V and ~0.16 V) when tested under otherwise the same conditions. A higher OCP value means a more favorable driving force for water oxidation since it determines the difference between the hole quasi-Fermi-level of the semiconductor heterojunction and the redox potential of the electrolyte. The above presented OCP result can be captured by the picture illustrated in Fig. 2b . For the pure BiVO 4 , the Fermi-level position of ideal BiVO 4 is close the valence band edge of BiVO 4 [9] , but the lattice defects formed during synthesis and surface state trapped electrons (V 4+ ) of pure BiVO 4 move the E f of pure BiVO 4 negatively (Supplementary Fig. 23 ) [38] , [39] , [40] . When the pure BiVO 4 photoanode was immersed in the solution, the E f of pure BiVO 4 became more negative than the redox potential due to Fermi-level pinning by surface trapped electrons, making the OCV dark of BiVO 4 relatively high [11] . Meanwhile, under AM 1.5 G illumination, the Fermi-level pinning effect prevented the E fn moving very close to the conduction band minimum (CBM) of BiVO 4 [11] , [38] , leading to a moderate OCV light and thus a low OCP (V ph ) of pure BiVO 4 very low. Importantly, the Mo doping in BiVO 4 could reduce the surface trap states and at the same time introduced new states, thus moderating the Fermi-level pinning effect (Supplementary Fig. 4 ) [41] . Due to the reduced Fermi-level pinning effect by Mo doping, for the 0.05% and 0.1% Mo-BiVO 4 photoanodes, the E f and E fn became more positive and negative than E f of the pure BiVO 4 photoanode, respectively, thereby enhancing the OCPs. However, for the 0.5% Mo-BiVO 4 , new states were introduced due to the excess Mo doping, and the E f became much closer to CBM, leading to high OCV dark (Supplementary Fig. 6 ) and thus a low OCP. As such, the OCP of 0.1% Mo-BiVO 4 is the best of all the samples we studied, in agreement with the corresponding PEC performance as will be presented below. As can be seen from Fig. 2a , the photocurrent density of 0.1% Mo-BiVO 4 reached 5.0 (±0.2) mA cm −2 at 1.23 V vs. RHE in solution with hole scavenger, which represents ~73% the theoretical water oxidation photocurrent density ( J max ) of BiVO 4 (6.8 mA cm −2 ). Thus the moderate Mo doping of BiVO 4 in the low end doping regime can increase the photo-voltage carrier concentration and mobility of the BiVO 4 photoanodes, and improve their onset potential and photocurrent density. Heterojunction engineering We now turn to our second strategy to optimize the PEC performance of BiVO 4 -based photoanodes by further increasing the utilization of J max . To accomplish it, we started with the basic C 3 N 4 /BiVO 4 junction, and then work up for optimization by B-doping C 3 N 4 and the Mo-doping BiVO 4 . Both LHE and charge separation have been enhanced, leading to the increase of J abs and Φ Sep of the photoanode. Supplementary Fig. 7 shows the UV–vis absorption spectra from the diffuse reflectance measurements and photographs of B-C 3 N 4 and C 3 N 4 . From visual inspection, the yellow color of B-C 3 N 4 is clearly deeper than C 3 N 4 , and correspondingly, the absorption of B-C 3 N 4 is also stronger than C 3 N 4 . From the plots in Supplementary Fig. 8a of (αhν) [2] vs. the photon energy (hν), the band-gap energy of C 3 N 4 and B-C 3 N 4 are 2.53 eV and 2.41 eV, respectively. Supplementary Fig. 8b is the LHE of B-C 3 N 4 /Mo-BiVO 4 , which exhibits stronger absorption in the range between 300 nm and 500 nm than Mo-BiVO 4 . Supplementary Fig. 8c shows the spectra of the solar irradiance of AM 1.5 G (ASTM G173-03) and those weighted by the LHE spectra of B-C 3 N 4 /Mo-BiVO 4 , which shows the J abs of B-C 3 N 4 /Mo-BiVO 4 achieved ~6.0 mA cm −2 . 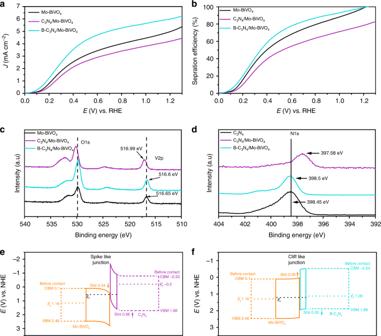Fig. 3 Photoelectrochemical performances and charge transfer processes.aLSV curves of C3N4/Mo-BiVO4, 0.1% Mo-BiVO4and B-C3N4/Mo-BiVO4measured at a scan rate of 25 mV s−1under AM 1.5 G irradiation in PPB solution with Na2SO3as a hole scavenger (pH 7).bSeparation efficiency (ΦSep) of C3N4/Mo-BiVO4, 0.1% Mo-BiVO4and B-C3N4/Mo-BiVO4. XPS core-level shifts ofcV 2p, O 1 s anddN 1 s. Schematic diagrams of the band structures ofeC3N4/Mo-BiVO4,fB-C3N4/Mo-BiVO4 Figure 3a compares the LSV curves of 0.1% Mo-BiVO 4 (black line), C 3 N 4 /Mo-BiVO 4 (cyan line) and B-C 3 N 4 /Mo-BiVO 4 (purple line) at a scan rate of 25 mV s −1 using 0.5 M Na 2 SO 3 as a hole scavenger in a PPB buffered aqueous solution (pH7) under AM 1.5 G irradiation. The photocurrent density of B-C 3 N 4 /Mo-BiVO 4 reached ~6 mA (±0.2) cm −2 at 1.23 V vs. RHE, and this is higher than that of 0.1% Mo-BiVO 4 (5 mA cm −2 ), at least partly due to the increase in LHE and J abs after the conjugation with B-C 3 N 4 . At 0.6 V vs. RHE, the photocurrent density of B-C 3 N 4 /Mo-BiVO 4 was 4.7 mA cm −2 , which is much higher than that of 0.1% Mo-BiVO 4 (3.4 mA cm −2 ). However, the photocurrent of C 3 N 4 /Mo-BiVO 4 only achieved 2.9 and 4.2 mA cm −2 at 0.6 and 1.23 V vs. RHE, which are lower than that of Mo-BiVO 4 (3.4 and 5 mA cm −2 ), although increased LHE and J abs by compositing C 3 N 4 and B-C 3 N 4 . The results of Φ Sep of Mo-BiVO 4 (black line), C 3 N 4 /Mo-BiVO 4 (cyan line) and B-C 3 N 4 /Mo-BiVO 4 (purple line) clearly shows that B-C 3 N 4 decoration can great increase the Φ Sep of Mo-BiVO 4 , while pure C 3 N 4 decoration will reduce the Φ Sep of Mo-BiVO 4 (Fig. 3b ). The Φ Sep of B-C 3 N 4 /Mo-BiVO 4 achieved 79 and 98% at 0.6 V and 1.23 V vs. RHE, respectively. The Φ Sep of B-C 3 N 4 /Mo-BiVO 4 at 0.6 V vs. RHE is higher than that of Mo-BiVO 4 (69%), and at 1.23 V vs. RHE, the Φ Sep of Mo-BiVO 4 andB-C 3 N 4 /Mo-BiVO 4 are achieved near 100% cause the charge separation of Mo-BiVO 4 and B-C 3 N 4 /Mo-BiVO 4 have reached their limits at higher bias voltage. However, the Φ Sep of C 3 N 4 /Mo-BiVO 4 only achieved 60 and 80% at 0.6 V and 1.23 V vs. RHE, which are even lower than that of Mo-BiVO 4 . This result shows that when C 3 N 4 is compositing the Mo-BiVO 4 , it has no effect on the separation of the photo-generated charges. These results mean that although the thermodynamic potential of pure C 3 N 4 and Mo-BiVO 4 are match, the heterojunction of pure C 3 N 4 and Mo-BiVO 4 became a compound center of photo-generated charge. Fig. 3 Photoelectrochemical performances and charge transfer processes. a LSV curves of C 3 N 4 /Mo-BiVO 4 , 0.1% Mo-BiVO 4 and B-C 3 N 4 /Mo-BiVO 4 measured at a scan rate of 25 mV s −1 under AM 1.5 G irradiation in PPB solution with Na 2 SO 3 as a hole scavenger (pH 7). b Separation efficiency ( Φ Sep ) of C 3 N 4 /Mo-BiVO 4 , 0.1% Mo-BiVO 4 and B-C 3 N 4 /Mo-BiVO 4 . XPS core-level shifts of c V 2p, O 1 s and d N 1 s. Schematic diagrams of the band structures of e C 3 N 4 /Mo-BiVO 4 , f B-C 3 N 4 /Mo-BiVO 4 Full size image As shown in Fig. 3c, d , when the Mo-BiVO 4 and pure C 3 N 4 are in contact, the O1s and V2p positive shift 0.34 eV and N1s negative shifts 0.96 eV. Supplementary Fig. 9 shows the CBM, VBM and Fermi level of BiVO 4 , Mo-BiVO 4, C 3 N 4 and B-C 3 N 4 by UPS and XPS VB spectra data (Supplementary Figs. 10 , 11 , 12 , and 13 ). The Fermi level of BiVO 4 and Mo-BiVO 4 are in the middle of their band gap (BiVO 4 : 1.21 eV and Mo-BiVO 4 : 1.16 eV) and the Fermi level of B-C 3 N 4 is close to its VBM, and the Fermi level of pure C 3 N 4 is close to its CBM. The DFT data confirms that the Fermi energy level of Mo-BiVO 4 and B-C 3 N 4 changed after Mo and B element doping (Supplementary Fig. 14 ). In detail, when Mo-BiVO 4 and C 3 N 4 come into contact to form a heterojunction, the bands on the two sides bend oppositely into the spike-like structure (Fig. 3e ), and thus the electrons from the C 3 N 4 side can hardly transfer to the Mo-BiVO 4 side. The holes inside Mo-BiVO 4 will hardly transfer to C 3 N 4 , as the existence of energy barrier at the interface. Therefore, the contact interface of pure C 3 N 4 and Mo-BiVO 4 will reduce the separation of photo-generated charges. On the other hand, due to the B element doping, the Fermi level of B-C 3 N 4 is getting closer to the VBM (Supplementary Fig. 9b ). As shown in Fig. 3d , when the Mo-BiVO 4 and B-C 3 N 4 are in contact, a cliff like junction is formed with the correct charge transfer direction, which will increase the separation of photo-generated charges. Supplementary Fig. 15 displays the Raman spectra of Mo-BiVO 4 , C 3 N 4 , B-C 3 N 4 , C 3 N 4 /Mo-BiVO 4 and B-C 3 N 4 /Mo-BiVO 4 . The Raman peaks at 702 cm −1 and 746 cm −1 are attributed to the C-N vibration of B-C 3 N 4 (Blue line). The peak at 816 cm −1 are attributed to the V–O vibration, while the peaks at 362 cm −1 and 323 cm −1 can be attributed to the VO 4 3- vibration of the Mo-BiVO 4 . The Raman peaks of B-C 3 N 4 (702 cm −1 , 746 cm −1 ) and Mo-BiVO 4 (362 cm −1 , 323 cm −1 ) shifted to 545 cm −1 , 620 cm −1 , and 340 cm −1 , 314 cm −1 in B-C 3 N 4 /Mo-BiVO 4 sample, indicating the formation of chemical bonds between B-C 3 N 4 and Mo-BiVO 4 . In other words, the B-C 3 N 4 is chemically linked to Mo-BiVO 4 . PEC water splitting performance In order to use the B-C 3 N 4 /Mo-BiVO 4 photoanode for PEC water splitting in solution without hole scavenger, the NiFeO x layer was used as an OEC material, which was deposited on the photo-active area of B-C 3 N 4 /Mo-BiVO 4 photoanode surface by photoelectrodeposition method. Supplementary Figs. 16 and 17 show the XPS data of Ni, N, B, C, Bi, Mo, O, and Fe. For B-doped C 3 N 4 , as can be seen from Supplementary Figs. 16c , the peak of B is located at around 191.9 eV, fairly close to the binding energy of B in the –C–N–B– and –N–B–(N) 2 – groups (192.1 eV) of the B-C 3 N 4 materials reported in the literature [42] . The oxidation state of B is consistent with the results of B-doped C 3 N 4 in the reported literature [27] . As shown in Fig. 4a and Supplementary Fig. 21 , the PEC water splitting capability of NiFeO x /B-C 3 N 4 /Mo-BiVO 4 photoanode (orange solid line) achieves 4.18 mA cm −2 and 5.93 (±0.3) mA cm −2 at 0.6 V vs. RHE and 1.23 V vs. RHE in PPB solution (pH 7), which are much higher than that of Mo-BiVO 4 photoanode and B-C 3 N 4 /Mo-BiVO 4 , Meanwhile, the photocurrent density of NiFeO x /B-C 3 N 4 /Mo-BiVO 4 photoanode at 0.6 V vs. RHE and 1.23 V vs. RHE are much close to that of NiFeO x /B-C 3 N/Mo-BiVO 4 photoanode (orange dotted line) in PPB solution with Na 2 SO 3 hole scavenger (pH 7, 4.37 (±0.3) mA cm −2 and 5.96 (±0.3) mA cm −2 ). Supplementary Fig. 18 shows that the B-C 3 N 4 can not only increase the photocurrent density in the low biased-voltage range (0.1~0.8 V vs. RHE) by increasing the separation efficiency of photoanode, but also increase the photocurrent density in the high biased-voltage range (0.8~1.3 V vs. RHE). The IPCEs of NiFeO x /B-C 3 N 4 /Mo-BiVO 4 , NiFeO x /Mo-BiVO 4 , NiFeO x / BiVO 4 , B-C 3 N 4 /Mo-BiVO 4 , Mo-BiVO 4 , and BiVO 4 at 0.54 V vs. RHE in PPB solution (pH 7), which shows that the B-C 3 N 4 can increase the charge separation efficiency and light absorption of photoanode. On the other hand, the NiFeO x cannot increase light absorption of photoanode, and it only plays the role of a co-catalyst (OEC) here (Supplementary Fig. 19 ). In Fig. 4b , due to the high oxygen evolution reaction capacity of NiFeO x OEC, the dark LSV of NiFeO x /B-C 3 N/Mo-BiVO 4 photoanode shows a remarkable cathodic shift (~340 mV) of onset potential compared to B-C 3 N 4 /Mo-BiVO 4 photoanode and Mo-BiVO 4 photoanode. However, the LSV curves of the B-C 3 N 4 /Mo-BiVO 4 and NiFeO x /B-C 3 N 4 /Mo-BiVO 4 recorded at a scan rate of 25 mV s −1 in PPB solution with Na 2 SO 3 as a hole scavenger (pH 7), which shows that the photocurrent density of samples measured in solution with Na 2 SO 3 will decline after the NiFeO x layer deposition (Supplementary Fig. 20 ). 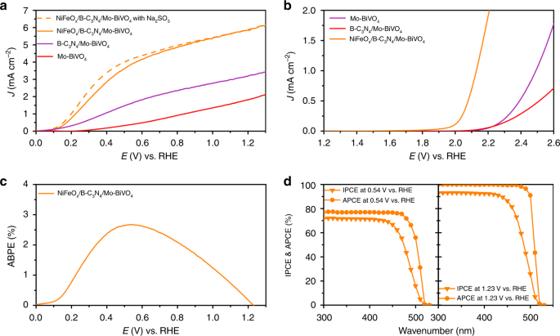Fig. 4 Photoelectrochemical performances. LSV curves of the Mo-BiVO4, B-C3N4/Mo-BiVO4and NiFeOx/B-C3N4/Mo-BiVO4recorded at a scan rate of 25 mV s−1in PPB solution without Na2SO3as a hole scavenger (pH 7)aunder AM 1.5 G irradiation andbin dark.cABPE of NiFeOx/B-C3N4/Mo-BiVO4.dIPCE and APCE of NiFeOx/B-C3N4/Mo-BiVO4at 0.54 V vs. RHE (left) and 1.23 V vs. RHE (right) in PPB solution (pH 7) Figure 4c shows the half-cell applied bias photo-to-current efficiency (ABPE) of the NiFeO x /B-C 3 N 4 /Mo-BiVO 4 photoanode. The ABPE is calculated to be 2.67% at 0.54 V vs. RHE, which is the highest recorded for BiVO 4 -based photoanodes (Fig. 6c ). Evidently, the highest efficiency has been achieved for the NiFeO x /B-C 3 N 4 /Mo-BiVO 4 photoanode at the lowest potential (0.54 V vs. RHE) among the previously reported values, which shows the highest performance of PEC water splitting for BiVO 4 -based photoanodes. Shown in Supplementary Figs. 25 and 26 are the LSV curves and ABPE measurement results in the two electrodes configuration (NiFeO x /B-C 3 N 4 /Mo-BiVO 4 photoanode and Pt cathode) in PPB solution (pH 7). It can be seen that the ABPE of whole PEC system (without reference electrode) achieved 2.1% at 0.62 V vs. Pt. Figure 4d shows the incident-photon-to-current conversion efficiency (IPCE) and the absorbed photon-to-current efficiency (APCE) spectra of NiFeO x /B-C 3 N 4 /Mo-BiVO 4 photoanode at 0.54 V vs . RHE and 1.23 V vs. RHE in PPB solution (pH 7). The maximum IPCE value of NiFeO x /B-C 3 N 4 /Mo-BiVO 4 photoanode reaches ~71 and 92% at 0.54 V vs. RHE and 1.23 V vs. RHE. The APCE of NiFeO x /B-C 3 N 4 /Mo-BiVO 4 photoanode reaches ~100% at 1.23 V vs. RHE, establishing the NiFeO x /B-C 3 N 4 /Mo-BiVO 4 photoanode used all the light it could absorb for PEC water splitting at 1.23 V vs. RHE. Therefore, these results clearly show that the NiFeO x OEC can greatly improve the PEC capacity of B-C 3 N 4 /Mo-BiVO 4 photoanode in the absence of any hole scavenger. Fig. 4 Photoelectrochemical performances. LSV curves of the Mo-BiVO 4 , B-C 3 N 4 /Mo-BiVO 4 and NiFeO x /B-C 3 N 4 /Mo-BiVO 4 recorded at a scan rate of 25 mV s −1 in PPB solution without Na 2 SO 3 as a hole scavenger (pH 7) a under AM 1.5 G irradiation and b in dark. c ABPE of NiFeO x /B-C 3 N 4 /Mo-BiVO 4 . d IPCE and APCE of NiFeO x /B-C 3 N 4 /Mo-BiVO 4 at 0.54 V vs. RHE (left) and 1.23 V vs. RHE (right) in PPB solution (pH 7) Full size image As shown in Fig. 5 and Supplementary Video 1 , the NiFeO x /B-C 3 N/Mo-BiVO 4 photoanode exhibits excellent operational stability for half-cell PEC water splitting in PPB solution (pH 7) at 0.54 V vs. RHE under AM 1.5 G irradiation. 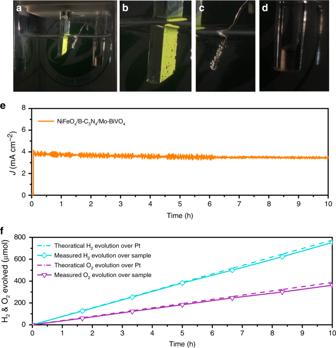Fig. 5 Photoelectrochemical water splitting performances. Photographs of the NiFeOx/B-C3N4/Mo-BiVO4photoanode in the PEC water splitting system (a), the NiFeOx/B-C3N4/Mo-BiVO4photoanode in a blown-up view (b), the Pt cathode (c), and the Ag/AgCl reference electrode (d).eChronoamperometry (i–t) curve of NiFeOx/B-C3N4/Mo-BiVO4photoanode collected at 0.54 V vs. RHE under AM 1.5 G illumination in PPB solution (pH 7).fH2and O2evolution of the NiFeOx/B-C3N4/Mo-BiVO4photoanode at 0.54 V vs. RHE; dashed curves indicate the H2and O2evolution with 98% Faraday efficiency 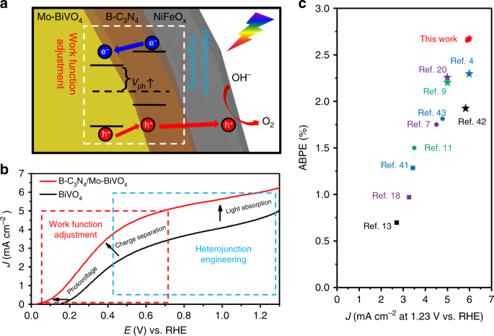Fig. 6 Photoelectrochemical water splitting characterization.aSchematic diagram illustrating the separation of photo-generated electrons and holes of the NiFeOx/B-C3N4/Mo-BiVO4photoanode,bLSV curves of pure-BiVO4, B-C3N4/Mo-BiVO4recorded at a scan rate of 25 mV s−1under AM 1.5 G one-sun irradiation in PPB solution using 0.5 M Na2SO3as a hole scavenger (pH 7),cspecific photocurrent density at 1.23 V vs. RHE and applied bias photo-to-current efficiency (ABPE) of BiVO4based photoanode4,7,9,11,13,18,20,41,42,43. Figure 5a shows the photograph of the NiFeO x /B-C 3 N/Mo-BiVO 4 photoanode half-cell PEC water splitting system, and Fig. 5b–d show the photographs of the photoanode, the Pt cathode and the Ag/AgCl reference electrode separately. The chronoamperometry curve of the NiFeO x /B-C 3 N 4 /Mo-BiVO 4 photoanode was collected at 0.54 V vs. RHE in 10 h. The photocurrent density of the NiFeO x /B-C 3 N 4 /Mo-BiVO 4 photoanode was initially 3.85 mA cm −2 and decreased by only 10% after 10 h of operation, demonstrating the good stability of the NiFeO x /B-C 3 N 4 /Mo-BiVO 4 photoanode during the long time irradiation in PPB solution (Fig. 5e ). And the photocurrent densities of the NiFeO x /Mo-BiVO 4 and NiFeO x /B-C 3 N 4 /Mo-BiVO 4 photoanodes decayed by 5 and 8% (Supplementary Fig. 24 ), respectively, very close to the stability testing result of the NiFeO x /B-C 3 N 4 /Mo-BiVO 4 photoanode at 0.54 V vs. RHE. These results confirm that the NiFeO x is a stable co-catalyst for the BiVO 4 -based photoanodes, essentially consistent with the recent reports. The generation rates of H 2 and O 2 by our half-cell system are measured to be 77.5 μM/h and 336 μm 33.6 μM/h, respectively, with Faradic efficiency of 98% (Fig. 5f ). Fig. 5 Photoelectrochemical water splitting performances. Photographs of the NiFeO x /B-C 3 N 4 /Mo-BiVO 4 photoanode in the PEC water splitting system ( a ), the NiFeO x /B-C 3 N 4 /Mo-BiVO 4 photoanode in a blown-up view ( b ), the Pt cathode ( c ), and the Ag/AgCl reference electrode ( d ). e Chronoamperometry (i–t) curve of NiFeO x /B-C 3 N 4 /Mo-BiVO 4 photoanode collected at 0.54 V vs. RHE under AM 1.5 G illumination in PPB solution (pH 7). f H 2 and O 2 evolution of the NiFeO x /B-C 3 N 4 /Mo-BiVO 4 photoanode at 0.54 V vs. RHE; dashed curves indicate the H 2 and O 2 evolution with 98% Faraday efficiency Full size image In conclusion, the NiFeO x /B-C 3 N 4 /Mo-BiVO 4 photoanode has provided an archetype to exploit the potential of boosting the photoelectrochemical performance by the synergistic combination of work function tuning and heterojunction construction. The bespoke photoanode achieved a remarkable photocurrent density of 3.85 mA cm −2 , ABPE of 2.67% and IPCE of 71% at 0.54 V vs. RHE, which are the highest yet reported with the lowest biased-voltage for BiVO 4 -based PEC materials. The NiFeO x /B-C 3 N/Mo-BiVO 4 photoanode exhibited significantly enhanced PEC activity for water splitting by systematically work function adjustment (Fig. 6a ). We have demonstrated the work function adjustment via Mo doping could reduce the interfacial energy loss and increase the open-circuit photo-voltage of BiVO 4 PEC cells. In addition, the creation and optimization of the heterojunction (p-n) of B-C 3 N 4 and Mo-BiVO 4 with correct charge transfer direction were accomplished by work function adjustment via B doping for C 3 N 4 , thereby increasing the separation of photo-generated electron-hole pairs at the B-C 3 N 4 and Mo-BiVO 4 interface (Fig. 6a, b ). The data of DFT calculation, XPS and UPS confirm the Fermi level and band shift of B-C 3 N 4 and Mo-BiVO 4 . This synergistic effect between B doping of C 3 N 4 and Mo doping of BiVO 4 with the NiFeO x OEC has allowed the NiFeO x /B-C 3 N 4 /Mo-BiVO 4 photoanode to achieve the record – the highest PEC water splitting performance (2.67% ABPE) with a fairly low bias-voltage (0.54 V vs. RHE), which shows the efficiency of ABPE are the highest recorded for BiVO 4 -based photoanodes [4] , [7] , [9] , [11] , [13] , [18] , [20] , [43] , [44] , [45] . The demonstration of the NiFeO x /B-C 3 N 4 /Mo-BiVO 4 photoanode with excellent PEC water splitting capability achieved by the synergistic combination of work function tuning and heterojunction deliberation will inform the design and development of the next-generation PEC materials and devices. Fig. 6 Photoelectrochemical water splitting characterization. a Schematic diagram illustrating the separation of photo-generated electrons and holes of the NiFeO x /B-C 3 N 4 /Mo-BiVO 4 photoanode, b LSV curves of pure-BiVO 4 , B-C 3 N 4 /Mo-BiVO 4 recorded at a scan rate of 25 mV s −1 under AM 1.5 G one-sun irradiation in PPB solution using 0.5 M Na 2 SO 3 as a hole scavenger (pH 7), c specific photocurrent density at 1.23 V vs. RHE and applied bias photo-to-current efficiency (ABPE) of BiVO 4 based photoanode [4] , [7] , [9] , [11] , [13] , [18] , [20] , [41] , [42] , [43] . Full size image Preparation of BiVO 4 and Mo-BiVO 4 electrode BiVO 4 photoanodes were fabricated by a two-step process via a modified method which was originally developed by Kim and Choi [7] . At first, a template-free electrochemical deposition was applied to prepare the BiOI nanosheets using a conventional three-electrode glass cell, where a piece of F-doped SnO 2 coated glass (FTO, Nippon Sheet Glass, 1 × 2 cm) served as the working electrode, a Pt electrode served as the counter electrode and an Ag/AgCl electrode served as the reference electrode. Generally, 50 mL of solution containing 0.4 M KI (99.0%, Tianjin Zhiyuan Reagent Co. Ltd.) and 0.04 M Bi(NO 3 ) 3 (99.0%, Shanghai Macklin Biochemical Co. Ltd) was adjusted pH to 1.7 by adding HNO 3 (65–68%, AR, Guangzhou Chemical Reagent). Then, 20 mL of absolute ethanol (100%) containing 0.23 M p-benzoquinone (97%, Aladdin) was mixed into the above solution and vigorously stirred for several minutes. Cathodic deposition of BiOI (1 × 1 cm area) was performed potentiostatically in the final solution at −0.1 V vs. Ag/AgCl at room temperature (RT) for 200 s. The second step was the conversion of BiOI to BiVO 4 . Dimethyl sulfoxide (DMSO, AR, Tianjin Damao Reagent) solution containing 0.2 M vanadyl acetylacetonate (VO(acac) 2 , 95%, Aladdin) was impregnated on BiOI electrodes (50 μL cm −1 ) and then annealed in air at 450 °C for 2 h with ramping rate of 2 °C min −1 . Lastly, the BiVO 4 electrodes were soaked in 1 M NaOH (AR, Guangzhou Chemical Reagent) solution for 1 h with gentle stirring to remove the excess V 2 O 5 . The obtained pure BiVO 4 electrodes were rinsed by deionizer water and dried at RT. Molybdenum doped BiVO 4 (Mo-BiVO 4 ) photoanodes were prepared in the same way by adding Na 2 MoO 4 as the Mo source. In detail, 1, 2, and 10 μL 0.1 M Na 2 MoO 4 (AR, Tianjin Damao Reagent) aqueous solution was added into 1 mL the above VO(acac) 2 DMSO solution before it was impregnated on BiOI electrodes. The corresponding concentration ratio of Mo/Bi was 0.05%, 0.1%, and 0.5%, respectively. Preparation of C 3 N 4 and B-C 3 N 4 The bulk graphite-C 3 N 4 (C 3 N 4 ) was fabricated by directly heating low-cost melamine (99%, Aladdin). In detail, 5 g melamine powder was placed in an alumina crucible with a cover, then heated to 500 °C for 2 h in a muffle furnace with a heating rate of 2 °C min −1 . The obtained bulk C 3 N 4 was grind into small powder, and 100 mg C 3 N 4 powder was dispersed in 100 mL isopropyl alcohol (AR, Tianjin Damao Reagent) and exfoliated by ultrasonication for 24 h to obtain C 3 N 4 nanosheets (C 3 N 4 -NS). The resultant dispersion was centrifuged at 3000 rpm for 10 min, and the supernatant containing exfoliated C 3 N 4 -NS was collected by pipette. Boron doped C 3 N 4 nanosheets (B-C 3 N 4 -NS) supernatants were prepared in the same way but heating the mixture of 0.5 g boric acid (GR, Aladdin) and 5 g melamine. Preparation of C 3 N 4 /BiVO 4 and B-C 3 N 4 /Mo-BiVO 4 electrode The BiVO 4 or Mo-BiVO 4 photoanodes were immersed into 20 mL C 3 N 4 -NS or B-C 3 N 4 -NS supernatants for 1 h. After rinsed with deionizer water, the obtained (B-)C 3 N 4 /(Mo-)BiVO 4 photoanodes were annealed at 350 °C in air for 1 h for better combination. Photoelectrodeposition of NiFeO x OEC layer NiFeO x OEC layer were synthesized using a simple photoelectrodeposition method reported. NiFeO x layer was photoelectrodeposited on the B-C 3 N 4 /Mo-BiVO 4 in 0.4 M FeSO 4 and 0.04 M NiSO 4 solution at 0.6 V vs. Ag/AgCl (total charge 100 mC/cm 2 ) at RT. The NiFeO x /B-C 3 N 4 /Mo-BiVO 4 electrode was then washed with deionizer water and dried in air at 60 °C. Analysis The as-synthesized products were characterized by a scanning electron microscope (SEM, Zeiss G-500), transmission electron microscopy (TEM, JEOL 2100 F, FEI Tecnai G 2 F30), X-Ray Diffractometer (XRD, D8 ADVANCE), X-ray Photoelectron Spectroscopy (XPS) and Ultroviolet Photoelectron Spectroscopy (UPS, Thermo Fisher Scientific ESCALab250) and Raman spectroscopy (Renishaw inVia). The optical properties of the products were measured with an UV–vis–NIR Spectrophotometer (UV–vis–NIR, Shimadzu UV-2450). Photoelectrochemical and electrochemical measurements All the PEC and electrochemical measurements were carried out in a three-electrode cell with a flat quartz window to facilitate illumination of the photoelectrode surface. The working electrode is the product fabricated in this work, while Pt electrode was used as a counter electrode and Ag/AgCl electrode was used as a reference electrode, respectively. The illumination source was AM 1.5 G solar simulator (Newport, LCS 100 94011 A (class A, Supplementary Fig. 29 ) directed at the quartz PEC cell (100 mW cm −2 ). Incident-photon-to-current conversion efficiency (IPCE) were collected by a Solartron 1280B electrochemical station with a solar simulator (Newport 69920, 1000 W xenon lamp), coupled with an infrared water filter (Oriel 6127) and aligned monochromator (Oriel Cornerstone 130 1/8 m). All the electrochemical measurements were performed on an SP-150 electrochemical workstation (SP-150, Bio-Logic SAS, France) at RT. More PEC and electrochemical calculations are shown in the Supporting information.